Direct isolation and RNA-seq reveal environment-dependent properties of engrafted neural stem/progenitor cells Neural stem/progenitor cell (NSPC) transplantation is a promising treatment for various neurodegenerative disorders including spinal cord injury, however, no direct analysis has ever been performed on their in vivo profile after transplantation. Here we combined bioimaging, flow-cytometric isolation and ultra-high-throughput RNA sequencing to evaluate the cellular properties of engrafted NSPCs. The acutely transplanted NSPCs had beneficial effects on spinal cord injury, particularly neuroprotection and neurohumoral secretion, whereas their in situ secretory activity differed significantly from that predicted in vitro . The RNA-sequencing of engrafted NSPCs revealed dynamic expression/splicing changes in various genes involved in cellular functions and tumour development depending on graft environments. Notably, in the pathological environment, overall transcriptional activity, external signal transduction and neural differentiation of engrafted NSPCs were significantly suppressed. These results highlight the vulnerability of engrafted NSPCs to environmental force, while emphasizing the importance of in situ analysis in advancing the efficacy and safety of stem cell-based therapies. As the adult central nervous system (CNS) has limited natural potential for repair and regeneration, spinal cord injury (SCI) causes permanent and severe motor/sensory dysfunctions, and currently available treatments are ineffective [1] , [2] , [3] . Therefore, the transplantation of stem cells such as neural stem/progenitor cells (NSPCs) is an exciting therapeutic option for replacing damaged neural cells and inducing functional recovery [3] , [4] , [5] , [6] , and some clinical trials have been performed [7] , [8] . However, the efficacy of NSPCs for treating SCI is currently insufficient, and unexpected serious side effects have been observed following NSPC transplantation [4] , [7] , [9] . More importantly, no direct analysis has ever been performed on the in vivo profile of NSPCs engrafted in injured spinal cord and thus the in vivo properties of engrafted cells still remain unclear. Therefore, the cellular mechanisms underlying functional improvement, the risk of tumorigenesis after transplantation and optimal transplantation protocols remains largely elusive [4] , [8] . Without assessing biological and molecular properties of engrafted cells in pathological environments, the development of effective and safe strategies for stem cell-based therapies cannot be possible. Here we evaluated the viability of transplanted NSPCs and their effects on neural apoptosis, inflammatory reactions and motor function after SCI to elucidate the in vivo activity of NSPCs. To directly assess the in vivo biology of engrafted NSPCs, we developed a combined method for isolating engrafted cells from the injured spinal cords and providing whole transcriptome information. Ultra-high-throughput RNA sequencing (RNA-seq) is a revolutionary tool for transcriptome profiling, which offers both single-base resolution for annotation and digital gene expression levels at the whole genome scale [10] , and overcomes several limitations of hybridization-based microarrays [10] , [11] . In particular, the wide dynamic range of RNA-seq allows robust capture of low-expression transcripts, including cytokines/chemokines, signal transduction molecules and transcriptional regulators [10] and direct comparisons of transcriptomes in different samples and under different conditions [10] , [12] . A detailed understanding of the cellular behaviour after transplantation is crucial to establish the efficacy and safety of stem cell-based therapies [4] , [5] , and our strategy will be applicable to various stem cell-based approaches. Cell viability and functional improvement We examined the engraftment and survival of NSPCs in mouse SCI using in vivo bioluminescent imaging (BLI) system. NSPCs were harvested from embryonic mouse striatum and labelled with luciferase and green fluorescent protein (GFP) reporter genes via lentiviral transduction, and GFP-positive cells were expanded with a neurosphere assay ( Supplementary Fig. S1 ). BLI detect transplanted cells expressing luciferase after the administration of the luciferase substrate, luciferin. This reaction depends on ATP and oxygen, and thus only living engrafted NSPCs can be noninvasively tracked in the same animal [13] . To examine whether the number of transplanted cells affects cell survival and functional improvement, different numbers of lentivirally labelled NSPCs (1×10 5 , 2.5×10 5 , 5×10 5 or 1×10 6 cells) were transplanted into the injured spinal cord immediately after contusion injury at the 10th thoracic level. After confirming that the number of transplanted NSPCs correlated with bioluminescence intensity, we tracked the bioluminescence intensity and observed comparable rates of NSPC survival, irrespective of the number of transplanted NSPCs ( Fig. 1a–c and Supplementary Fig. S1 ). In all groups, bioluminescence intensity largely decreased during the first week after transplantation in line with previous histopathological studies [14] , [15] , [16] . This would be due to the apoptotic and necrotic cell death [17] . Although these cell deaths could be caused by immune rejection [18] , significant T-cell infiltration, which is an indicator of immune rejection, was not observed at the initial and late phase after transplantation ( Supplementary Fig. S2 ). Because our model consisted of a C57BL6 syngeneic allograft, little graft rejection response would occur in this study. No increases in the bioluminescence intensity, indicator of tumorigenesis, were observed within the experimental period. All NSPC-transplanted groups showed better locomotor function recovery than the medium-injected control group in two open-field motor scores (Basso, Beattie and Bresnahan (BBB) score and Basso Mouse Scale (BMS)) and footprint analysis ( Fig. 1d and Supplementary Fig. S3a,b ). However, functional recovery was not significantly different among the NSPC-transplanted groups. Also, cell fate was not significantly affected by the number of transplanting NSPCs ( Supplementary Fig. S3c–f ). Correlational analysis revealed no relationship between the number of surviving NSPCs and the subsequent functional recovery at any time point in 74 NSPC-transplanted mice ( Fig. 1e and Supplementary Fig. S3g ). Moreover, bioluminescence intensities and motor scores at 4, 7 and 42 days after transplantation (DAT) were comparable among the NSPC-transplanted mice that were divided into two groups based on motor scores or bioluminescence intensities at 42 DAT ( Fig. 1f,g ), indicating the effects of NSPC transplantation on functional recovery to be saturated at a specific number of cells. Furthermore, we transplanted a broader range of NSPCs (ranging from 2.5×10 4 to 2.5×10 6 cells). The transplantation of 2.5×10 4 NSPCs did not significantly affect functional improvement, but that of 2.5×10 6 NSPCs made the injury worse by eliciting a robust inflammatory reaction ( Supplementary Fig. S4 ), resulting in a negative effect on functional improvement ( Fig. 1h and Supplementary Movies 1–3 ). These results indicate that an optimal number of transplanted cells are beneficial to SCI. 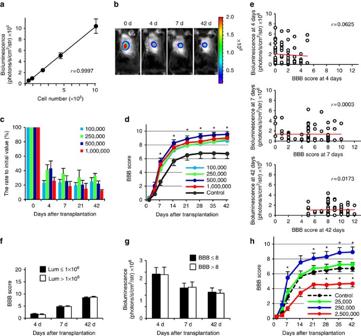Figure 1: Number of transplanted/surviving NSPCs and functional recovery. (a) Correlation between the number of transplanted NSPCs and the bioluminescence intensity measuredin vivoimmediately after transplantation (P<0.01, Pearson correlation coefficient). (b) Images of a representative mouse transplanted with 5×105NSPCs, confirming long-term cell viability. (c) Time course of the rate of bioluminescence intensity relative to the initial value over a period of 6 weeks after transplantation in each NSPC-transplanted group (1×105cells (n=14), 2.5×105cells (n=17), 5×105cells (n=22) and 1×106cells (n=21). (d) Time course of functional recovery as determined by the BBB scores of control group (n=21) and each NSPC-transplanted group. (e) Functional recovery and bioluminescent intensity revealed no significant correlations at any time point (P=0.62 (4 DAT);P=0.54 (7 DAT); andP=0.89 (42 DAT), Pearson correlation coefficient). (f) Retrospective comparison of functional recovery between NSPC-transplanted mice with bioluminescent intensities >1×106(n=30) and less (n=44) at 42 DAT. (g) Retrospective comparison of bioluminescent intensities between NSPC-transplanted mice with BBB score >8 (n=39) and less (n=35) at 42 DAT. (h) Time course of functional recovery on BBB score in NSPC-transplanted group (2.5×104cells (n=13), 2.5×105cells (n=13), 2.5×106cells (n=13) and control group (n=14)). *P<0.05 versus control, ANOVA with Tukey–Kramerpost-hoctest. Data are represented as mean±s.e.m. Figure 1: Number of transplanted/surviving NSPCs and functional recovery. ( a ) Correlation between the number of transplanted NSPCs and the bioluminescence intensity measured in vivo immediately after transplantation ( P <0.01, Pearson correlation coefficient). ( b ) Images of a representative mouse transplanted with 5×10 5 NSPCs, confirming long-term cell viability. ( c ) Time course of the rate of bioluminescence intensity relative to the initial value over a period of 6 weeks after transplantation in each NSPC-transplanted group (1×10 5 cells ( n =14), 2.5×10 5 cells ( n =17), 5×10 5 cells ( n =22) and 1×10 6 cells ( n =21). ( d ) Time course of functional recovery as determined by the BBB scores of control group ( n =21) and each NSPC-transplanted group. ( e ) Functional recovery and bioluminescent intensity revealed no significant correlations at any time point ( P =0.62 (4 DAT); P =0.54 (7 DAT); and P =0.89 (42 DAT), Pearson correlation coefficient). ( f ) Retrospective comparison of functional recovery between NSPC-transplanted mice with bioluminescent intensities >1×10 6 ( n =30) and less ( n =44) at 42 DAT. ( g ) Retrospective comparison of bioluminescent intensities between NSPC-transplanted mice with BBB score >8 ( n =39) and less ( n =35) at 42 DAT. ( h ) Time course of functional recovery on BBB score in NSPC-transplanted group (2.5×10 4 cells ( n =13), 2.5×10 5 cells ( n =13), 2.5×10 6 cells ( n =13) and control group ( n =14)). * P <0.05 versus control, ANOVA with Tukey–Kramer post-hoc test. Data are represented as mean±s.e.m. Full size image Neuroprotective effects of engrafted NSPCs There are several possible explanations for NSPC-mediated functional improvement after SCI, such as synapse formation by graft-derived neurons, remyelination by graft-derived oligodendrocytes, growth support, neuroprotection and immunomodulation [4] , [5] , [19] . To determine which mechanism mainly contributes to functional improvement in acute transplantation, we evaluated the weekly recovery in the open-field score and observed the most prominent effect within the first week after transplantation ( Fig. 2a ). In this study, we therefore focused on the actions and effects of engrafted NSPCs within 7 DAT. In this phase, engrafted NSPCs did not yet differentiate because they did not express any neuronal or glial markers, but were positive for Nestin, a marker of undifferentiated NSPCs ( Fig. 2b ). These results indicate the functional improvement in this phase to be mainly due to either neuroprotective and/or immunomodulatory effects, rather than cell replacement or growth support, which requires much more time. During this time period, significant increases in the expression levels of several neurotrophic factors were observed, including nerve growth factor, glial cell-derived neurotrophic factor (GDNF), brain-derived neurotrophic factor (BDNF), ciliary neurotrophic factor (CNTF), insulin-like growth factor 1 (IGF1), hepatocyte growth factor (HGF), platelet-derived growth factor (PDGF) a, PDGFb and vascular endothelial growth factor a (VEGFa), in the NSPC-transplanted groups ( Fig. 2c and Supplementary Fig. S5a,b ). These expression levels increased in proportion to the number of transplanted cells, indicating in vivo neurohumoral secretion by the engrafted NSPCs ( Supplementary Fig. S5c ). 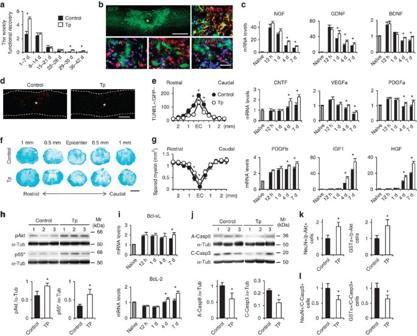Figure 2: NSPCs prevent the activation of the mitochondrial apoptosis pathway. (a) Weekly recovery as assessed by BBB score of NSPC-transplanted group (Tp;n=74) and control group (n=21, *P<0.05 versus control, ANOVA with Bonferronipost-hoctest.) (b) Immunohistochemical analysis of engrafted NSPCs at 7 DAT. Asterisk indicates the lesion epicentre. Scale bar, 1 mm and 50 μm. (c) Time course of gene expression levels (normalized to naïve spinal cord) of neurotrophic factors as determined by qPCR (n=8 per group, *P<0.05 versus control, Mann–WhitneyU-test). (d) TUNEL staining of sagittal section at 7 DAT in both the mice transplanted with 5×105NSPCs (Tp) and control. Asterisk indicates the lesion epicentre. Scale bar, 1 mm. (e) Quantification of TUNEL positive cells on axial sections 7 DAT (Tp:n=9; control:n=8 per group, *P<0.05 versus control, Student'st-test). (f) Luxol Fast Blue (LFB) staining of axial sections at 7 DAT. Scale bar, 1 mm. (g) Quantification of the area of LFB-positive spared myelin 7 DAT (Tp:n=9; control:n=8 per group, *P<0.05 versus control, Student'st-test). (h) Western blot analysis of activated Akt and NF-κB using antibodies that specifically recognize the activated form (phospho-Akt (pAkt) or phospho-NF-κB p65 (p65*)). (n=8 per group, *P<0.05 versus control, Mann–WhitneyU-test). (i) Gene expression of anti-apoptosis proteins (Bcl-2 and Bcl-xL) was significantly increased 7 DAT in the NSPC-transplanted group (n=8 per group, *P<0.05 versus control, Mann–WhitneyU-test). (j) Western blot analysis of activated caspase 9 (A-Casp9) and cleaved caspase 3 (C-Casp3). (n=8 per group, *P<0.05 versus control, Mann–WhitneyU-test). (k) Comparison of the number of phospho-Akt and NeuN or GSTπ double-positive cells (n=5 per group, Mann–WhitneyU-test). (l) Comparison of the number of C-Casp3 and NeuN or GSTπ double-positive cells (n=5 per group, *P<0.05 versus control, Mann–WhitneyU-test). Data are represented as mean±s.e.m. Figure 2: NSPCs prevent the activation of the mitochondrial apoptosis pathway. ( a ) Weekly recovery as assessed by BBB score of NSPC-transplanted group (Tp; n =74) and control group ( n =21, * P <0.05 versus control, ANOVA with Bonferroni post-hoc test.) ( b ) Immunohistochemical analysis of engrafted NSPCs at 7 DAT. Asterisk indicates the lesion epicentre. Scale bar, 1 mm and 50 μm. ( c ) Time course of gene expression levels (normalized to naïve spinal cord) of neurotrophic factors as determined by qPCR ( n =8 per group, * P <0.05 versus control, Mann–Whitney U -test). ( d ) TUNEL staining of sagittal section at 7 DAT in both the mice transplanted with 5×10 5 NSPCs (Tp) and control. Asterisk indicates the lesion epicentre. Scale bar, 1 mm. ( e ) Quantification of TUNEL positive cells on axial sections 7 DAT (Tp: n =9; control: n =8 per group, * P <0.05 versus control, Student's t -test). ( f ) Luxol Fast Blue (LFB) staining of axial sections at 7 DAT. Scale bar, 1 mm. ( g ) Quantification of the area of LFB-positive spared myelin 7 DAT (Tp: n =9; control: n =8 per group, * P <0.05 versus control, Student's t -test). ( h ) Western blot analysis of activated Akt and NF-κB using antibodies that specifically recognize the activated form (phospho-Akt (pAkt) or phospho-NF-κB p65 (p65*)). ( n =8 per group, * P <0.05 versus control, Mann–Whitney U -test). ( i ) Gene expression of anti-apoptosis proteins (Bcl-2 and Bcl-xL) was significantly increased 7 DAT in the NSPC-transplanted group ( n =8 per group, * P <0.05 versus control, Mann–Whitney U -test). ( j ) Western blot analysis of activated caspase 9 (A-Casp9) and cleaved caspase 3 (C-Casp3). ( n =8 per group, * P <0.05 versus control, Mann–Whitney U -test). ( k ) Comparison of the number of phospho-Akt and NeuN or GSTπ double-positive cells ( n =5 per group, Mann–Whitney U -test). ( l ) Comparison of the number of C-Casp3 and NeuN or GSTπ double-positive cells ( n =5 per group, * P <0.05 versus control, Mann–Whitney U -test). Data are represented as mean±s.e.m. Full size image Because these neurohumoral factors prevent neural apoptosis by the activation of the PI3K-Akt/NF-κB signalling pathway in vitro [20] , [21] , [22] , [23] , the neuroprotective effects through NSPC transplantation were examined. Histopathological examinations at 7 DAT revealed fewer TUNEL-positive cells and more spared myelin in the NSPC-transplanted group ( Fig. 2d–g ). Furthermore, we observed the activation of Akt and NF-κB (p65) ( Fig. 2h ), and a significant upregulation of their downstream transcriptional targets, Bcl-2 and Bcl-xL [20] , [23] ( Fig. 2i ), at 7 DAT in the NSPC-transplanted group, resulting in decreased activation of caspases 9 and 3 ( Fig. 2j ). To identify the cells that showed decreased apoptosis after transplantation, immunohistochemical analysis was performed 7 DAT. Increased Akt activation and decreased caspase-3 activation was observed in neurons and oligodendrocytes ( Fig. 2k,l and Supplementary Fig. S6 ). In addition to neuroprotective effects, NSPCs are known to have immunomodulative effects [4] , [19] , [24] ; therefore, the acute inflammatory response after NSPC transplantation was also examined. Although increased expression of anti-inflammatory cytokines, such as interleukin (IL)-10 and transforming growth factor beta 1 (TGF-β1) was observed, no significant differences were observed in terms of the expression of pro-inflammatory cytokines or the number of infiltrating inflammatory cells ( Fig. 3a–f ). Consistently, Fas, FasL and caspase 8 expression levels, the extrinsic apoptotic-cascade mediators induced by inflammation, and caspase 8 activation did not significantly differ from that in the controls ( Fig. 3g,h ). These results indicate that engrafted NSPCs ameliorate pathological changes during the acute phase of SCI, particularly the secondary damage cascades that are dependent on the mitochondrial apoptosis pathway. 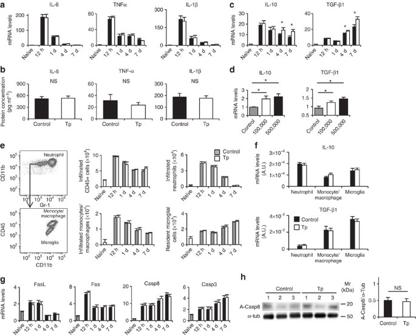Figure 3: The inflammatory reaction following NSPC transplantation. (a) The mRNA levels of anti-inflammatory cytokines between control and 5×105NSPC-transplanted group (n=8 per group). There were no significant differences at any time points between the two groups. (b) The comparison of pro-inflammatory cytokine concentrations at 12 h measured by ELISA (n=4 per group). (c) The mRNA levels of anti-inflammatory cytokines by qPCR (n=8 per group). There was significant increase of anti-inflammatory cytokines after 4 DAT in transplanted groups compared with control groups. *P<0.05 versus control by Mann–WhitneyU-test. (d) The expression levels of anti-inflammatory cytokines increased in 1×105and 5×105NSPC-transplanted mice at 4 DAT (n=5 per group). The mRNA levels were normalized to injured spinal cord of the control at 4 days (*P<0.05 versus control by ANOVA with Dunnettpost-hoctest). (e) Each population of inflammatory cells was analysed by flow cytometry from a pool of CD45posi inflammatory cells obtained from injured spinal cord, neutrophils: CD11bhigh/Gr-1posi, monocytes/ macrophages: CD45high/CD11bposi/Gr-1nega-int, and microglia: CD45int/CD11bposi/Gr-1nega-int. The absolute numbers of infiltrated inflammatory cells were comparable between two groups at each time point (n=15 per group). (f) The expression levels of IL-10 and TGF-b1 in each sorted inflammatory population at 4 DAT. (g) The mRNA levels of extrinsic apoptotic pathway mediaters by qPCR (n=6–8 per group). (h) Western blot analysis for activated caspase 8 (A-Casp8) (n=6 per group). Data are represented as mean±s.e.m. Figure 3: The inflammatory reaction following NSPC transplantation. ( a ) The mRNA levels of anti-inflammatory cytokines between control and 5×10 5 NSPC-transplanted group ( n =8 per group). There were no significant differences at any time points between the two groups. ( b ) The comparison of pro-inflammatory cytokine concentrations at 12 h measured by ELISA ( n =4 per group). ( c ) The mRNA levels of anti-inflammatory cytokines by qPCR ( n =8 per group). There was significant increase of anti-inflammatory cytokines after 4 DAT in transplanted groups compared with control groups. * P <0.05 versus control by Mann–Whitney U -test. ( d ) The expression levels of anti-inflammatory cytokines increased in 1×10 5 and 5×10 5 NSPC-transplanted mice at 4 DAT ( n =5 per group). The mRNA levels were normalized to injured spinal cord of the control at 4 days (* P <0.05 versus control by ANOVA with Dunnett post-hoc test). ( e ) Each population of inflammatory cells was analysed by flow cytometry from a pool of CD45posi inflammatory cells obtained from injured spinal cord, neutrophils: CD11bhigh/Gr-1posi, monocytes/ macrophages: CD45high/CD11bposi/Gr-1nega-int, and microglia: CD45int/CD11bposi/Gr-1nega-int. The absolute numbers of infiltrated inflammatory cells were comparable between two groups at each time point ( n =15 per group). ( f ) The expression levels of IL-10 and TGF-b1 in each sorted inflammatory population at 4 DAT. ( g ) The mRNA levels of extrinsic apoptotic pathway mediaters by qPCR ( n =6–8 per group). ( h ) Western blot analysis for activated caspase 8 (A-Casp8) ( n =6 per group). Data are represented as mean±s.e.m. Full size image Flow-cytometric isolation of engrafted NSPCs To assess whether the increased expression of neurohumoral factors was attributed to engrafted NSPCs, we tried to isolate engrafted NSPCs from the injured spinal cord. After digesting and dissociating spinal cord tissues into single cells, the GFP-positive engrafted NSPCs were purified by flow cytometry (fluorescence-activated cell sorting: FACS) ( Fig. 4a,b ). Approximately 1.1×10 5 cells were collected at 7 DAT (mean: 112,663±8,122 cells, n =5) from the injured spinal cord transplanted with 5×10 5 NSPCs (collection rate: 91.5±17.3%) and RNA was prepared from FACS-purified NSPCs. Gene expression levels in NSPCs were not altered by FACS manipulation ( Fig. 4c ). The expression of neurohumoral factors was observed in FACS-purified NSPCs by reverse transcription PCR (RT–PCR) ( Fig. 4d ). These results were confirmed by immunostaining using the VEGFa or BDNF antibody, in situ hybridization using PDGFa, PDGFb or IGF1 probes with GFP staining, and the laser-capture microdissection method 7 DAT of histopathological sections ( Supplementary Fig. S7 ). Changes in their expression properties, such as a gradual increase in differentiation-related genes, as well as a decrease in stemness markers, ruled out the possibility that only a single specific population survived and was isolated by our procedure ( Fig. 4e ). The gene expression profiles of several neurohumoral factors significantly differed between the FACS-purified and pre-transplantation NSPCs ( Fig. 4d–g ). Almost all secretory activities significantly increased in FACS-purified NSPCs at 7 DAT compared with those in NSPCs at 7 days in vitro (DIV; Fig. 4f–h ). These results indicate that the graft environment greatly affects the secretory activities of engrafted cells. 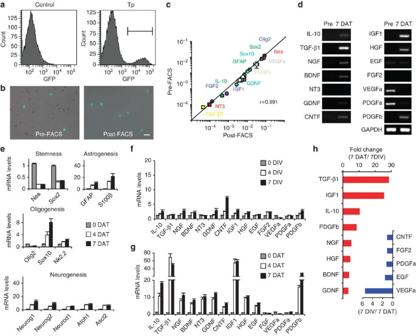Figure 4: Direct isolation and gene expression analysis of engrafted NSPCs. (a) FACS analysis for the homogenate of injured spinal cord tissue at 7 DAT. The GFP+ population was only observed in the homogenate of NSPC-transplanted spinal cords. (b) Imaging of isolated NSPCs from the injured spinal cord before and after FACS. Scale bar, 50 μm. (c) Gene expression levels of NSPCs were not altered by the FACS procedure (r=0.991,P<0.01;n=3 per group, Pearson correlation coefficient). (d) Compared with the pre-transplantation NSPCs (Pre), semiquantitative RT–PCR revealed increased expressions ofIl10, tgfb1, ngf, bdnf, gdnf, cntf, igf1, hgf,andpdgfb, whereas decreased expressions ofpdgfa andvegfain FACS-purified NSPCs transplanted into injured spinal cord at 7 DAT. (e) Time course of the gene expressions of the stemness and differentiation in isolated NSPCs from injured spinal cord (n=9 per time point). (f,g) Time course of the gene expressions of neurohumoral factors in NSPCs cultured for 4 and 7 DIV (f), and those in NSPCs isolated from injured spinal cord at 4 and 7 DAT (g) (n=9 per time point). Gene expression levels were normalized to pre-transplantation NSPCs. (h) Comparison of gene expression levels of neurohumoral factors in NSPCs after 7 daysin vitroandin vivo. Bar graph indicates fold changes of increased (red) and decreased (blue) gene expression in engrafted NSPCs (7 DAT) compared with cultured NSPCs (7 DIV) as assessed by qPCR. Data are represented as mean±s.e.m. Figure 4: Direct isolation and gene expression analysis of engrafted NSPCs. ( a ) FACS analysis for the homogenate of injured spinal cord tissue at 7 DAT. The GFP+ population was only observed in the homogenate of NSPC-transplanted spinal cords. ( b ) Imaging of isolated NSPCs from the injured spinal cord before and after FACS. Scale bar, 50 μm. ( c ) Gene expression levels of NSPCs were not altered by the FACS procedure ( r =0.991, P <0.01; n =3 per group, Pearson correlation coefficient). ( d ) Compared with the pre-transplantation NSPCs (Pre), semiquantitative RT–PCR revealed increased expressions of Il10, tgfb1, ngf, bdnf, gdnf, cntf, igf1, hgf, and pdgfb , whereas decreased expressions of pdgfa a nd vegfa in FACS-purified NSPCs transplanted into injured spinal cord at 7 DAT. ( e ) Time course of the gene expressions of the stemness and differentiation in isolated NSPCs from injured spinal cord ( n =9 per time point). ( f,g ) Time course of the gene expressions of neurohumoral factors in NSPCs cultured for 4 and 7 DIV ( f ), and those in NSPCs isolated from injured spinal cord at 4 and 7 DAT ( g ) ( n =9 per time point). Gene expression levels were normalized to pre-transplantation NSPCs. ( h ) Comparison of gene expression levels of neurohumoral factors in NSPCs after 7 days in vitro and in vivo . Bar graph indicates fold changes of increased (red) and decreased (blue) gene expression in engrafted NSPCs (7 DAT) compared with cultured NSPCs (7 DIV) as assessed by qPCR. Data are represented as mean±s.e.m. Full size image RNA-seq of NSPCs To elucidate environmental influences on the cellular properties of NSPCs, RNA-seq was performed on NSPCs in four different contexts: pre-transplantation NSPCs (Pre), NSPCs grown for 7 days in a culture dish (in dish), in naïve spinal cord (in naïve) or in injured spinal cord (in injured). The quality of RNA prepared from FACS-purified NSPCs was excellent and comparable across all samples ( Fig. 5a ). Eight sequencing libraries were constructed (two samples from each NSPC population) and sequenced on a giga-sequencer; the sequenced fragments were mapped to the mouse reference genome using TopHat and assembled with Cufflinks [25] . More than 21 million 36-base sequence reads were obtained, of which >83% were aligned and included >11,000 genes from a single library ( Supplementary Table S1 ). The median expression level of the reconstructed mRNA was estimated by fragments per kilobase of exonic sequences per million aligned reads (FPKM) [11] . Biological replicates for different samples gave extraordinary identical genome-wide translational profiles ( Fig. 5b ), confirming the accuracy and precision of our RNA-seq analysis. RNA-seq profiling was validated using quantitative PCR (qPCR; Fig. 5c ). Consistent with qPCR data ( Fig. 4f–h ), RNA-seq data showed higher TGF-β1 expression and lower VEGFa expression in NSPCs in naïve and in injured compared with other contexts ( Fig. 5d ). The expression differences of each neurotrophic factor in Fig. 4f–h were also confirmed by RNA-seq ( n =3; Supplementary Fig. S8 ). Overall, the expression of large sets of genes varied considerably, and several environment-dependent salient genes were identified ( Fig. 5e ). The Venn diagram summarizes the overlapping transcripts detected in each sample ( Fig. 5f ). Furthermore, considerable differences were observed in the expression levels of nearly two-thirds of the genes between NSPCs in dish versus those in naïve or in injured (>2-fold change; Fig. 5g ). These results highlight molecular variability of NSPCs depending on the environment and the importance of in situ analysis of engrafted cells. 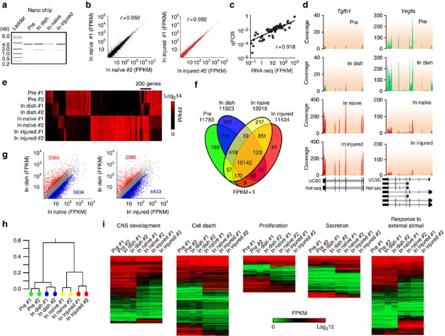Figure 5: RNA sequencing of NSPCs in different contexts. (a) RNA libraries were constructed from NSPCs under four different contexts. RNA integrity of NSPCs was determined using an Agilent 2100 Bioanalyzer. (b) Biological replicates ofin vivosamples. A very strong correlation was observed between NSPCs in naïve sample #1 and #2 (r=0.959,P<0.01, Pearson correlation coefficient), and also between NSPCs in injured sample #1 and #2 (r=0.992,P<0.01, Pearson correlation coefficient). (c) Validation of RNA-seq data by qPCR with 63 known transcripts. RNA-seq data strongly correlated with qPCR data (r=0.991,P<0.01, Pearson correlation coefficient). (d) Visualization of expression data forTgfb1andVegfa. Wiggle plots directly represent the number of each individual read. (e) Gene expression heatmap showing several environment-dependent salient genes. (f) The Venn diagram showing the number of overlapping transcripts (FPKM >1) detected in each context. (g) Scatter plots between NSPCs in dish and NSPCs in naïve or in injured. These represent many differentially expressed genes with more than twofold (in red) or less than half (in blue). (h) Hierarchical clustering of NSPCs in the four contexts. NSPC populations were clearly distinguished whether they were inin vivoorin vitroenvironments. (i) Heatmaps depicting gene expression changes of NSPCs in terms of the environment regarding to CNS development (273 genes), cell death (305 genes), proliferation (140 genes), secretion (218 genes) and response to external stimuli (426 genes). Molecular profiles of NSPCs vary considerably betweenin vitroandin vivo. Figure 5: RNA sequencing of NSPCs in different contexts. ( a ) RNA libraries were constructed from NSPCs under four different contexts. RNA integrity of NSPCs was determined using an Agilent 2100 Bioanalyzer. ( b ) Biological replicates of in vivo samples. A very strong correlation was observed between NSPCs in naïve sample #1 and #2 ( r =0.959, P <0.01, Pearson correlation coefficient), and also between NSPCs in injured sample #1 and #2 ( r =0.992, P <0.01, Pearson correlation coefficient). ( c ) Validation of RNA-seq data by qPCR with 63 known transcripts. RNA-seq data strongly correlated with qPCR data ( r =0.991, P <0.01, Pearson correlation coefficient). ( d ) Visualization of expression data for Tgfb1 and Vegfa . Wiggle plots directly represent the number of each individual read. ( e ) Gene expression heatmap showing several environment-dependent salient genes. ( f ) The Venn diagram showing the number of overlapping transcripts (FPKM >1) detected in each context. ( g ) Scatter plots between NSPCs in dish and NSPCs in naïve or in injured. These represent many differentially expressed genes with more than twofold (in red) or less than half (in blue). ( h ) Hierarchical clustering of NSPCs in the four contexts. NSPC populations were clearly distinguished whether they were in in vivo or in vitro environments. ( i ) Heatmaps depicting gene expression changes of NSPCs in terms of the environment regarding to CNS development (273 genes), cell death (305 genes), proliferation (140 genes), secretion (218 genes) and response to external stimuli (426 genes). Molecular profiles of NSPCs vary considerably between in vitro and in vivo . Full size image Comparison of the global gene expression levels with hierarchical clustering showed that NSPC populations were clearly distinguished based on whether they were in vivo NSPCs (in naïve and in injured) or in vitro NSPCs (Pre and in dish) ( Fig. 5h ). To distinguish the biological properties of in vivo NSPCs from in vitro NSPCs, in silico analyses of the RNA-seq data were performed. A transcription factor-binding site (TFBS) enrichment analysis [26] identified ten over-represented TFBSs in the in vivo and in vitro NSPCs, respectively ( P <0.0001; Supplementary Fig. S9 ). The gene expression levels of the transcription factors corresponding with over-represented TFBSs were examined using RNA-seq and qPCR. Immunoregulatory and metabolic transcription factors, such as Nfkb1 , Rela and Pparg, were over-regulated in in vivo NSPCs, whereas the growth-, proliferation- and differentiation-related transcription factors, such as Pax6 , Myc , Bmyc , Maz , Egr1 , Egr2 , Creb1 , Creb3 and Creb5, were over-regulated in in vitro NSPCs ( Supplementary Fig. S9 ), suggesting different transcriptional regulation patterns between the two groups. Gene ontology (GO) analysis, which classifies abundant gene expression data into functional categories and provides biological interpretations [27] , revealed 79 GO terms, such as the response to external stimuli, regulation of apoptosis and cytokine production, to be significantly over-represented in in vivo NSPCs, whereas 56 GO terms, including neurogenesis, RNA biosynthesis and reproductive developmental processes were significantly over-represented in in vitro NSPCs ( Supplementary Figs S10 and S11 ). These results indicate that engrafted NSPCs develop graft environment-dependent properties that cannot be precisely predicted before transplantation in terms of several cellular functions, including cell differentiation, survival, proliferation, secretory activities and response to external stimuli ( Fig. 5i ). Differences in NSPCs engrafted in naïve and injured spinal cord To investigate the biological differences between NSPCs engrafted in normal physiological versus pathological environment, the profiles of NSPCs in naïve and in injured were compared. RNA-seq demonstrated considerable differences in nearly one-third of the expressed genes (FPKM>2-fold change) and almost all these genes were downregulated in NSPCs in injured compared with NSPCs in naïve ( Fig. 6a ). Similarly, the transcriptional activity, which was indicated by read counts, decreased across the entire genome in NSPCs transplanted in injured spinal cords ( Fig. 6b ). These data indicating repressed transcriptional activities under the pathological environment were further confirmed by qPCR ( Fig. 6c ). In GO analysis, we found 22 GO terms, including biological metabolic processes and intracellular component biosynthesis, to be significantly over-represented in NSPCs transplanted in injured spinal cord, whereas 33 GO terms, such as the response to external stimuli, cell proliferation, cell adhesion and nerves system development, were over-represented in NSPCs transplanted in naïve spinal cord ( Fig. 6d,e ). These results were contrary to our expectations because the response to external stimuli of engrafted NSPCs was assumed to be strongly upregulated in the injured spinal cord owing to the inflammatory milieu with abundant signalling ligands. However, these data indicate that the external signal transduction was significantly suppressed in the engrafted NSPCs in the pathological environment. The relative ranking method was used to confirm these results. All expressed genes were arranged in the descending order in each sample and the relative ranks of genes with this function to the expressed genes were compared between NSPCs in naïve and in injured. Individual gene rank values with this function were largely lower in NSPCs in injured ( Fig. 6f ) and several genes encoding signal transduction molecules were downregulated in almost every signalling pathway in these NSPCs ( Fig. 6g ). Transcriptional repression was also observed in differentiation-associated genes in NSPCs transplanted in injured spinal cords ( Fig. 7a ). Consistent with gene expression data, only a few differentiated NSPCs were observed in injured spinal cords, although numerous engrafted NSPCs differentiated in naïve spinal cords 14 DAT ( Fig. 7b,c ). Because their differentiation was observed at 42 DAT in both environments ( Fig. 7d ), these results revealed that the neural differentiation of transplanted NSPCs is hindered in injured spinal cords. Contrary to the results of signal transduction and differentiation, survival-associated genes were generally activated in NSPCs in injured than that in naïve ( Fig. 7e ) and the Bcl-2/Bax ratio, which is a key determinant in cell death/survival [28] , was significantly higher in NSPCs in injured than that in naïve ( Fig. 7f,g ). These results of an anti-apoptotic state in NSPCs transplanted in injured spinal cord indicate that engrafted NSPCs can adequately survive in the injured niche by regulating survival-associated genes without the influence of transcriptional repression. Actually, BLI revealed no significant differences in the overall survival rate at 7 DAT ( Fig. 7h ) and comparable levels of apoptotic NSPCs were noted with TUNEL staining ( Fig. 7i ). 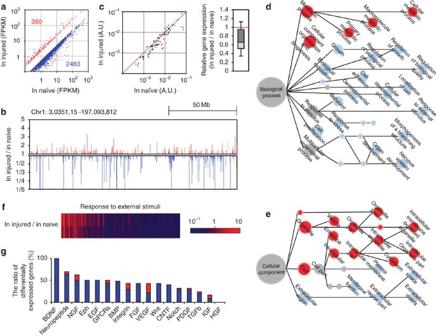Figure 6: Transcriptome analysis of engrafted NSPCs from naive and injured spinal cord. (a) Scatter plots of gene expression levels (FPKM) revealing significant differences between NSPCs in injured and in naïve. The expression levels of 380 genes were >2-fold (in blue) and of 2483 were <0.5-fold (in red) in NSPCs in injured. (b) Differences in expression intensity (read count) per 100 kb on chromosome 1 between NSPCs in injured and in naive. This graph shows the ratio of read counts in NSPCs transplanted in injured spinal cords to read counts in NSPCs transplanted in naïve spinal cords. (c) Validation of the transcriptional repression in NSPCs engrafted in injured spinal cord by qPCR with 96 randomly selected genes (P<0.001, Pearson correlation coefficient). (d,e) Gene ontology map showing significantly over-represented GO terms in NSPCs in injured compared with in naïve (in red) and NSPCs in naïve compared with in injured (in blue) (adjustedP-value <0.001, Fisher's exact test with Benjamini–Hochberg correction). (f) Heatmap depicting differences in the relative rank values of individual genes with the GO term 'response to external stimuli' (473 genes). Lower values (<1) tend to be blue, whereas higher values (>1) tend to be red in NSPCs in injured compared with in naive. The genes in NSPCs in injured were largely ranked lower than those NSPCs in naïve. (g) Ratio of upregulated (red) or downregulated (blue) genes (>1.5-fold change) to the total genes in each signalling pathway in NSPCs in injured compared with NSPCs in naïve. Figure 6: Transcriptome analysis of engrafted NSPCs from naive and injured spinal cord. ( a ) Scatter plots of gene expression levels (FPKM) revealing significant differences between NSPCs in injured and in naïve. The expression levels of 380 genes were >2-fold (in blue) and of 2483 were <0.5-fold (in red) in NSPCs in injured. ( b ) Differences in expression intensity (read count) per 100 kb on chromosome 1 between NSPCs in injured and in naive. This graph shows the ratio of read counts in NSPCs transplanted in injured spinal cords to read counts in NSPCs transplanted in naïve spinal cords. ( c ) Validation of the transcriptional repression in NSPCs engrafted in injured spinal cord by qPCR with 96 randomly selected genes ( P <0.001, Pearson correlation coefficient). ( d,e ) Gene ontology map showing significantly over-represented GO terms in NSPCs in injured compared with in naïve (in red) and NSPCs in naïve compared with in injured (in blue) (adjusted P -value <0.001, Fisher's exact test with Benjamini–Hochberg correction). ( f ) Heatmap depicting differences in the relative rank values of individual genes with the GO term 'response to external stimuli' (473 genes). Lower values (<1) tend to be blue, whereas higher values (>1) tend to be red in NSPCs in injured compared with in naive. The genes in NSPCs in injured were largely ranked lower than those NSPCs in naïve. ( g ) Ratio of upregulated (red) or downregulated (blue) genes (>1.5-fold change) to the total genes in each signalling pathway in NSPCs in injured compared with NSPCs in naïve. 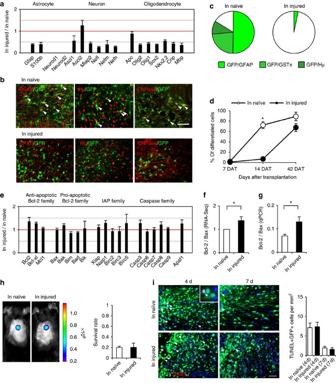Figure 7: Differentiation and survival of NSPCs transplanted into naïve and injured spinal cord. (a) Fold changes (in injured/in naïve) in the expression levels of differentiation-associated genes as determined by RNA-seq (n=3 per group). (b) Immunohistochemical analysis of NSPCs transplanted into naïve spinal cord and injured spinal cord at 14 DAT. GFAP, Hu or CNPase+ differentiated NSPCs were observed (arrow head) in naïve spinal cord but injured spinal cord. Scale bar, 100 μm. (c) Percentage of GFAP, Hu or CNPase/ GFP double-positive NSPCs to total GFP-positive NSPCs in naïve and injured spinal cord at 14 DAT. (d) Fold changes (in injured/in naïve) in the expression levels of survival-associated genes as determined by RNA-seq (n=3 per group). (e,f) The bcl-2/bax expression ratio in engrafted NSPCs as determined by RNA-seq (f;n=3 per group) and qPCR (g;n=5 per group). (h) Rate of bioluminescence intensity at 7 DAT relative to the initial value were comparable between NSPCs in naïve and in injured (n=6 per group). (i) Triple staining with TUNEL (red), GFP (green) and Hoechst (blue) show TUNEL+ NSPCs at 4 DAT, but few TUNEL+ NSPCs were observed at 7 DAT in either environment. Inset shows apoptotic NSPCs at higher magnification (arrow head). Asterisk indicates the injected site. The number of TUNEL+/GFP+ cells were comparable at 4 and 7 DAT between NSPCs transplanted into naïve and injured spinal cord (n=5 per group). Scale bar, 50 μm. *P<0.05 compared with naïve, Mann–WhitneyU-test. Data are represented as mean±s.e.m. Full size image Figure 7: Differentiation and survival of NSPCs transplanted into naïve and injured spinal cord. ( a ) Fold changes (in injured/in naïve) in the expression levels of differentiation-associated genes as determined by RNA-seq ( n =3 per group). ( b ) Immunohistochemical analysis of NSPCs transplanted into naïve spinal cord and injured spinal cord at 14 DAT. GFAP, Hu or CNPase+ differentiated NSPCs were observed (arrow head) in naïve spinal cord but injured spinal cord. Scale bar, 100 μm. ( c ) Percentage of GFAP, Hu or CNPase/ GFP double-positive NSPCs to total GFP-positive NSPCs in naïve and injured spinal cord at 14 DAT. ( d ) Fold changes (in injured/in naïve) in the expression levels of survival-associated genes as determined by RNA-seq ( n =3 per group). ( e,f ) The bcl-2/bax expression ratio in engrafted NSPCs as determined by RNA-seq ( f ; n =3 per group) and qPCR ( g ; n =5 per group). ( h ) Rate of bioluminescence intensity at 7 DAT relative to the initial value were comparable between NSPCs in naïve and in injured ( n =6 per group). ( i ) Triple staining with TUNEL (red), GFP (green) and Hoechst (blue) show TUNEL+ NSPCs at 4 DAT, but few TUNEL+ NSPCs were observed at 7 DAT in either environment. Inset shows apoptotic NSPCs at higher magnification (arrow head). Asterisk indicates the injected site. The number of TUNEL+/GFP+ cells were comparable at 4 and 7 DAT between NSPCs transplanted into naïve and injured spinal cord ( n =5 per group). Scale bar, 50 μm. * P <0.05 compared with naïve, Mann–Whitney U -test. Data are represented as mean±s.e.m. Full size image As tumorigenesis is closely associated with abnormal gene expression and/or alternative splicing of pro-oncogenes [29] , [30] , [31] , the representative pro-oncogenes in the CNS were quantified [32] , [33] . We observed significant expressions of such pro-oncogenes in NSPCs and differences between the two in Igf2r , pdgfrb, Hif1a, Fos , Smo , Idh1 , Pax6 and Olig2 ( Fig. 8a ). The dynamic range of RNA-seq facilitates the assessment of almost all genes involved in the glioma development/growth pathway depicted in the Kyoto encyclopaedia of genes and genomes (KEGG) [34] ( Fig. 8b ), suggesting our combined method to be feasible for evaluating tumour initiating potential of engrafted cells. Several brain tumour-specific alternative splicing variants (skipping or increased/decreased expression in specific exons) were also identified in the genes of NSPCs in injured [31] , [35] ( Fig. 8c and Supplementary Fig. S12 ). Moreover, distinct splicing variants were identified in Mcl-1 , which has longer and shorter isoforms that are formed by skipping the second exon [35] , [36] . The longer gene product of Mcl-1 L, which is involved in tumorigenesis [36] , was dominant in NSPCs in injured, whereas Mcl-1S, the shorter one, was the main product in NSPCs in naive ( Fig. 8d ). The differential expression of the splicing variants was confirmed by RT–PCR ( Fig. 8e,f ). These results indicate a possible increase in the degree of malignancy for engrafted cells in pathological environments. 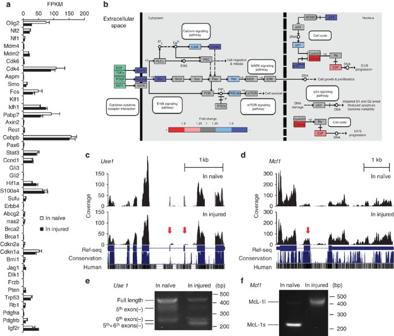Figure 8: Expression variability of tumour-related genes in engrafted NSPCs. (a) Absolute expression levels and differences in pro-oncogenes associated with CNS tumorigenesis (n=3 per group). (b) The pathological environment significantly affected the expression level of each mediator involved in the KEGG glioma pathway. The average expression level ofCdk6were >1.5-fold higher, whereas those ofEgfr,Pdgfra,Shc2, Camk2aandCdkn2awere <1.5-fold lower in NSPCs in injured than that in NSPCs in naïve (n=3 per group). (c,d) Wiggle plots showing the coverage of each exon for (c)Use1and (d)Mcl-1.Arrows indicate the exon with different splicing frequencies between the two. (e,f) Differences in the splice variant frequency inUse1(e) andMcl-1(f) as determined by RT–PCR. Figure 8: Expression variability of tumour-related genes in engrafted NSPCs. ( a ) Absolute expression levels and differences in pro-oncogenes associated with CNS tumorigenesis ( n =3 per group). ( b ) The pathological environment significantly affected the expression level of each mediator involved in the KEGG glioma pathway. The average expression level of Cdk6 were >1.5-fold higher, whereas those of Egfr , Pdgfra , Shc2, Camk2a and Cdkn2a were <1.5-fold lower in NSPCs in injured than that in NSPCs in naïve ( n =3 per group). ( c,d ) Wiggle plots showing the coverage of each exon for ( c ) Use1 and ( d ) Mcl-1. Arrows indicate the exon with different splicing frequencies between the two. ( e,f ) Differences in the splice variant frequency in Use1 ( e ) and Mcl-1 ( f ) as determined by RT–PCR. Full size image In this study, flow-cytometric isolation and RNA-seq were used to investigate the in vivo profile of engrafted NSPCs. Using this method, we found the biological properties of engrafted NSPCs, including the risk of malignancies, to be dynamically altered depending on their environment. Notably, overall transcriptional activity, external signal transduction and neural differentiation were significantly suppressed in NSPCs transplanted into injured spinal cords, emphasizing the need for in situ analysis to establish safe and effective stem cell-based therapies. Furthermore, using BLI, we demonstrated the presence of an appropriate range in the number of transplanting cells for SCI. In clinical trials, the transplantation protocols are completely different and, in particular, the number of transplanted cells varies considerably, which is also true in animal studies [5] , [7] , [8] . This hampers the establishment of an optimal treatment for SCI. In this study, we demonstrated that the transplantation of an excessive number of cells inversely prevented functional recovery following SCI, which emphasizes the need to define the optimal protocols to maximize their efficacy for clinical trials. The mechanisms underlying functional improvement remain unclear, which also present a significant hurdle for clinical translation of stem cell-based therapy for SCI [4] . Although engrafted NSPCs could facilitate functional recovery after SCI through multiple mechanisms [4] , [5] , [8] , our results revealed that neuroprotective effect is most significant for acute phase of SCI. Furthermore, we directly confirmed the neurohumoral secretion of engrafted NSPCs and demonstrated their secretory activities to be mostly enhanced after transplantation. Of the secreted neurohumoral substances, PDGF, IGF, TGF-β1 and IL-10 have critical roles in preventing neural apoptosis via the PI3K-Akt/NF-κB pathway [20] , [21] , [22] , [37] . Nerve growth factor and BDNF prevent activation of the mitochondrial apoptotic pathway via the P75NTR-mediated NF-κB pathway [23] , [38] . NF-κB activation induces the upregulation of anti-apoptotic genes, including Bcl-2 and Bcl-xL [20] , [23] and the Akt pathway could independently block the mitochondrial apoptotic pathway [23] . We demonstrated the activation of these mitochondrial apoptotic cascades following SCI to be attenuated by NSPC transplantation, providing a reasonable neuroprotective mechanism due to several neurohumoral factors. Expression microarrays are most widely used for transcriptome analysis; however, it is difficult to capture genes that are expressed at low levels, such as cytokine/chemokine, differentiation factors, signal transduction molecules and transcription factors, due to their narrow dynamic range and high background signals [10] . In contrast, RNA-seq can capture genes with low expression levels in a digital manner [10] and is therefore particularly useful for elucidating cellular activities, such as secretion, differentiation, signal transduction and transcriptional regulation. This technology highlights the graft environment-dependent properties of engrafted NSPCs and their vulnerability to environmental changes. The neural development of NSPCs was significantly inhibited in vivo , particularly in the injured spinal cord, indicating the reduction of their differentiation potential after transplantation. Moreover, under DNA damage-inducible conditions, mammalian cells repress transcriptional activities for self-defense and attenuate their response to environmental influences to resist disruptive external forces [39] , [40] . We found that engrafted NSPCs developed these specialized stress responses when transplanted into injured spinal cords, providing a plausible explanation for the persistence of undifferentiated engrafted NSPCs for an extended period of time [41] and failure of external manipulation. These results highlight the difficulty in obtaining cells that differentiate into the desired lineage in vivo and the need for innovative strategies that can overcome the environmental factors to improve the efficacy of stem cell-based therapies. One major obstacle of stem cell-based therapy is the risk of tumorigenesis [4] , [5] . Recently, Amariglio et al . [42] reported that transplanted NSPCs gave rise to glioneuronal neoplasms in a patient with ataxia telangiectasia. Although this report is controversial [43] , [44] , this highlights one of the biggest safety hurdles to overcome. Although NSPCs are tissue-derived stem cells that are unlikely to develop tumours [43] , all mammalian cells can turn into tumour cells caused by DNA damage, and the damage to the genes occurs by chance following various genotoxic insults [29] , [30] . Acute inflammation can contribute to tumour initiation by inducing DNA damage through reactive oxygen/nitrogen species, and chronic inflammation is a major cause of malignancy in many tumours [30] . Following SCI, cellular inflammation is excessive during the acute phase and it persists for a long time [2] , [45] . Thus, the risk of tumour initiation of transplanted cells would be increased in injured spinal cords. Actually, a positive correlation between traumatic injury and development of malignancy has recently been reported in the CNS [42] . To support this insight, RNA-seq demonstrated that NSPCs are exposed to various types of stress that could lead to DNA damage after transplantation [2] . Furthermore, RNA-seq can provide information about not only gene expression but also gene structure, such as splicing variants [25] . Therefore, our strategy enabled a direct and exhaustive analysis of complex transcriptomes, including the splicing variants responsible for tumorigenesis after transplantation [31] , [46] . In this study, we observed that brain tumour-specific alternative splicing increased in NSPCs transplanted in injured spinal cords than those transplanted in naïve spinal cords [31] . In addition, we found that expression levels of the longer isoform of Mcl-1, which is a prognostic and predictive marker for tumour development [35] , [36] , significantly increased in NSPCs in injured spinal cords. These results indicate that the risk of tumour initiation of transplanted cells increased in injured spinal cords. Because the graft environment is potentially related to the risk of tumour development of transplanted cells, an in situ analysis of transplanted cells will be needed to ensure the safety of stem cell-based therapies for patients. Studies on stem cell-based therapy focused enhancing their efficacy by genetic modification. Our findings, however, strongly indicate the importance of precisely assessing the reciprocal actions between engrafted cells and the pathological environment to ensure the efficacy and safety of the cells. Our methods, findings, and transcriptome databases contribute to advancing stem cell-based therapies for the treatment of SCI and other CNS disorders. A better understanding of the in situ behaviour of engrafted cells and developing a solid experimental basis for each pathological condition are required for there to be progress toward the successful clinical application of stem cell-based therapies. Primary culture and lentiviral transduction of NSPCs Methods for the culture and expansion of NSPCs have been described previously [13] . Briefly, the striatum of C57BL6 or BALBc mice on embryonic day 14 was mechanically dissociated, and concentrated lentiviruses were added into the culture medium to infect the primary NSPCs. Lentiviral vector expressing both luciferase and GFP was generated in 293T cells by transient transfection of the transfer vectors pCSII-EF-Luc-IRES2-Venus, pLP1, pLP2 and pLP/VSVG (Invitrogen) using GeneJuice Transfection Reagent (Novagen), followed by ultracentrifugation and titration, as described previously [13] . After the purification of GFP-positive transfected cells by FACS and passaged two times in a media hormone mix supplemented with 2% B27 (Invitrogen), 20 ng ml −1 FGF-2 and 20 ng ml −1 EGF (Peprotech), neurospheres were used for transplantation and analysis. For the in vitro assay, neurospheres were plated onto poly- L -lysine-coated cover slips and allowed to differentiate for 7 DIV. For RNA-seq experiments, NSPCs were harvested from the embryonic striatum of commercially available green mice (Japan SLC) and expanded and cultured with the same method. Bioluminescence imaging Bioluminescence image was performed using the Xenogen-IVIS 50-cooled CCD optical macroscopic imaging system (SC BioScience) following a previously published protocol [13] . All images were analysed with Igor (WaveMetrics) and Living Image software (Xenogen). SCI and cell transplantation Adult female C57BL6 mice were anesthetized via an intraperitoneal injection of sodium pentobarbital (somnopentyl; 50 mg kg −1 ). SCI was induced using Infinite Horizons Impactor at 70 kilodyne on 10th thoracic level [47] . A 25-μl Hamilton syringe (Hamilton) with a glass tip was inserted into the epicentre of the injured spinal cord and 2 μl of the cell suspension was injected at 0.5 μl min −1 using a stereotaxic injector (KDS 310; Muromachi-kikai). Control animals only received 2 μl conditioned medium [13] . At the over-dose experiment, 4 μl of cell suspension or conditioned medium was injected into injured spinal cords of each group. Motor functions were evaluated with a locomotor open-field rating scale on the BBB score [13] and the Basso Mouse Scale [47] . Footprint analysis was performed only on mice scored as frequently or consistently plantar stepping at 42 days after SCI. All animal studies were approved by the Committee of Ethics on Animal Experiment in Faculty of Medicine, Kyushu University. Experiments were conducted in accordance with the institutional guidelines and regulations for animal experiments. Flow cytometry and cell sorting For analysis of the infiltrated inflammatory cells, the spinal cord samples (4-mm long) were dissociated in collagenase (Invitrogen) and stained with antibodies, as previously described [47] , followed by analysis using FACSAria II flow cytometer and FACSDiva software (BD Biosciences). Phycoerythrin-Cy7 (PE-Cy7)-conjugated CD45 (1:10), fluorescein isothiocyanate-conjugated CD11b (1:10), PE-conjugated Gr-1 (1:50) and biotin-conjugated Nk1.1 (1:10) antibodies were used to examine myeloid cell infiltration. Allophycocyanin (APC)-conjugated streptavidin (1:10) was added to label the biotin-conjugated antibodies. PE-Cy7-conjugated CD45 (1:10), APC-conjugated CD3 (1:10), PE-conjugated CD4 (1:10) and fluorescein isothiocyanate-conjugated CD8 (1:10) antibodies were used to examine T-cell infiltration. All antibodies were purchased from eBioscience. For the isolation of engrafted NSPCs, the dissected spinal cord samples (4-mm long) were minced with scissors and then digested in 0.5% Trypsin with 0.5 mg ml −1 DNase for 5 min at 37 °C. The digests were further dissociated by gentle pipetting with a plastic pipette. The cell suspension was washed in Dulbecco's modified Eagle's medium and filtered through a 50-μm nylon cell strainer to isolate any tissue debris. The single-cell suspension was collected by centrifugation and resuspended in FACS buffer and propidium iodide was added to determine cell viability and then analysed with FACSAria II. Recollection rate was estimated from the BLI data; the number of GFP-positive cells recollected by FACS was divided by the estimated number of surviving cells using the BLI measurements. Immunohistochemistry and immunoblotting After the mice were transcardially fixed with 4% paraformaldehyde, the spinal cord was removed, dehydrated and embedded in an OCT compound [47] . The frozen sections were cut in the sagittal plane at 14 μm or axial plane at 20 μm. For immunostaining, the sections were stained with primary antibodies to NeuN, Hu, APC-CC1, GSTπ, GFAP, Nestin, phospho-Akt or cleaved caspase 3. For TUNEL staining, an ApopTag red in situ kit (Chemicon) was used. The number of TUNEL+/GFP− cells was counted in axial sections at 500 μm intervals and the number of TUNEL+/GFP+ cells was counted in sagittal sections at 280-μm intervals. Luxol Fast Blue staining was performed to calculate the area of spared myelin as described previously [47] . For immunoblotting, the following antibodies were used for: activated caspase 9, cleaved caspase 3, phospho-Akt, phospho-p65 (Ser536) and α-tubulin. All antibodies used are described in Supplementary Methods . Enzyme-linked immunosorbent assay (ELISA) assays were performed using the IL-6, IL-1β, and TNF-α ELISA kit (Bender Medsystems) [47] . Quantification methods are detailed in Supplementary Methods . Quantitative and semiquantitative RT–PCR Total RNA was isolated from the spinal cord (4-mm long) or inflammatory cells using RNeasy Lipid Tissue or Mini Kit (Qiagen). For complementary DNA (cDNA) synthesis, the reverse transcriptase reaction was performed using PrimeScript first-strand cDNA Synthesis Kit (Takara Bio). qPCR was performed using primers specific to the genes of interest ( Supplementary Table S2 ) and SYBR Premix Dimmer Eraser (Takara Bio). Data were normalized to glyceraldehyde-3-phosphate dehydrogenase. qPCR was performed in triplicate [47] . In situ hybridization with GFP staining The spinal cord was dissected after its perfusion, fixed with Tissue Fixative (Genostaff), and then embedded in paraffin, and sectioned at 6 μm. For in situ hybridization, as a first staining, tissue sections were de-waxed, rehydrated, fixed with 4% paraformaldehyde and then treated with 10 μg ml −1 proteinase K in phosphate-buffered saline for 30 min at 37 °C. Hybridization was performed with probe ( Supplementary Table S3 ) at a concentration of 300 ng ml −1 in the Probe Diluent (Genostaff) at 60 °C for 16 h. After hybridization, the sections were treated with 50% formamide, followed by incubation with RNAse. After blocking, they were incubated with anti-DIG AP-conjugated antibody (1:1,000, Roche) for 2 h. Colouring reactions were performed with NBT/BCIP solution (Sigma-Aldrich) overnight. For immunohistochemistry as a second staining after in situ hybridization, endogenous peroxidase was blocked with 0.3% H 2 O 2 for 30 min, followed by incubation with Protein Block (Dako) and a avidin/biotin blocking kit (Vector). The sections were incubated with an anti-GFP rabbit polyclonal antibody (Invitrogen). They were incubated with biotin-conjugated goat anti-rabbit Ig (Dako), followed by the addition of peroxidase-conjugated streptavidin (Nichirei). Peroxidase activity was visualized by diaminobenzidine. The sections were mounted with CC/Mount (DBS). Laser-capture microdissection At 7 DAT, fresh injured spinal cords were immediately frozen in dry ice/hexane and stored in a deep freezer at −80 °C. The tissues were sectioned into 10-μm thick slices using a cryostat at −20 °C and mounted on PEN membrane slides. Sections were then fixed in ice-cold acetone for 2 min. GFP-positive and -negative cells were dissected with a LMD 6500 system (Leica Microsystems GmbH) and transferred by gravity into a microcentrifuge tube cap placed directly beneath the section. The tube cap was filled with 75 μl of RLT buffer (Qiagen). For each sample, cells that were dissected from one series of sagittal sections, each separated by 140 mm, from an individual animal were used. Total RNA was isolated using the RNeasy Micro Kit (Qiagen). RNA-sequencing for NSPCs Construction of the libraries, mapping fragments to the genome, transcript assembly, abundance estimation and data analysis are described in Supplementary Information . All sequencing data from this study are available at the DNA Data Bank of Japan Sequence Read Archive under submission ID: DRA000217. Statistical analysis Statistical analyses were performed using the two-tailed unpaired Student's t -test, Mann–Whitney U -test for single comparisons, and one-way factorial analysis of variance (ANOVA) or two-way repeated measures ANOVA followed by the post-hoc Bonferroni, Dunnett or Tukey–Kramer correction for multiple comparisons. Correlational analyses were performed using the Pearson correlation coefficient. In all statistical analyses, significance was defined as P <0.05. How to cite this article: Kumamaru, H. et al . Direct isolation and RNA-seq reveal environment-dependent properties of engrafted neural stem/progenitor cells. Nat. Commun. 3:1140 doi: 10.1038/ncomms2132 (2012).